Tracking the Atlantic Multidecadal Oscillation through the last 8,000 years Understanding the internal ocean variability and its influence on climate is imperative for society. A key aspect concerns the enigmatic Atlantic Multidecadal Oscillation (AMO), a feature defined by a 60- to 90-year variability in North Atlantic sea-surface temperatures. The nature and origin of the AMO is uncertain, and it remains unknown whether it represents a persistent periodic driver in the climate system, or merely a transient feature. Here, we show that distinct, ∼ 55- to 70-year oscillations characterized the North Atlantic ocean-atmosphere variability over the past 8,000 years. We test and reject the hypothesis that this climate oscillation was directly forced by periodic changes in solar activity. We therefore conjecture that a quasi-persistent ∼ 55- to 70-year AMO, linked to internal ocean-atmosphere variability, existed during large parts of the Holocene. Our analyses further suggest that the coupling from the AMO to regional climate conditions was modulated by orbitally induced shifts in large-scale ocean-atmosphere circulation. The Atlantic multidecadal oscillation (AMO) has been identified as a coherent pattern of oscillatory changes in North Atlantic sea-surface temperature (SST) with a period of about 60–90 years [1] , [2] . Indices of the AMO have traditionally been based on average annual SST anomalies in the North Atlantic region [3] . To account for the influence of the recent global warming trend on North Atlantic SST, revised AMO indices have subsequently been defined by including global mean SSTs [4] , [5] ( Fig. 1 ). 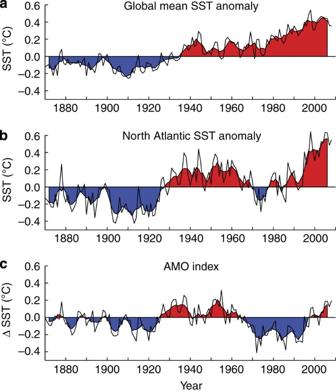Figure 1: Global and North Atlantic climate trends over the past∼150 years. (a) Global annual mean sea-surface temperature (SST) anomalies from HadISST for the period 1870–2008 (Ref.58)(thin black line). (b) Annual mean North Atlantic SST anomalies for the period 1870–2008 (ref.58; thin black line). (c) The Atlantic multidecadal oscillation (AMO) index for the period 1870–2008. The modern AMO index4is defined by subtracting the global mean SST anomalies (a) from the North Atlantic SST anomalies (b). Five-year running means are shown by heavy black lines with fill in all panels. Figure 1: Global and North Atlantic climate trends over the past ∼ 150 years. ( a ) Global annual mean sea-surface temperature (SST) anomalies from HadISST for the period 1870–2008 (Ref. 58 )(thin black line). ( b ) Annual mean North Atlantic SST anomalies for the period 1870–2008 (ref. 58 ; thin black line). ( c ) The Atlantic multidecadal oscillation (AMO) index for the period 1870–2008. The modern AMO index [4] is defined by subtracting the global mean SST anomalies ( a ) from the North Atlantic SST anomalies ( b ). Five-year running means are shown by heavy black lines with fill in all panels. Full size image The idea that slow changes in ocean circulation influence climate variability in the North Atlantic region goes back half a century [6] . Today, we have several lines of evidence suggesting that SST variations related to the AMO drive climate and precipitation patterns over North America [7] , [8] , [9] , droughts in the Sahel region of Africa [10] , variability in Northeast Brazilian rainfall [11] , and tropical hurricane frequency and intensity [12] . The AMO is also believed to influence regional to hemispheric-scale climate trends as far away as the Tibetan Plateau and India [13] , possibly through changes in the interhemispheric redistribution of heat [2] . However, because the instrumental SST records only span ∼ 150 years, it remains a matter of debate whether the observed SST variability merely reflects a transient feature on a 'red noise' background or a truly oscillatory phenomenon [14] , [15] . Answering this question requires a longer perspective that extends significantly further back in time. Studies of corals [14] , tree rings [16] , estuarine fossil pigments [17] and sea-spray in Greenland ice cores [18] indicate that a 60- to 100-year oscillation was also present in the North Atlantic region during the latest centuries preceding the instrumentally observed AMO. However, the available evidence for a pre-industrial AMO remains inconclusive. These oscillatory climate variations have been attributed to internal variability of the ocean related to changes in the Meridional overturning circulation [1] , [19] , a notion that has been supported by numerical studies showing that SST is the primary carrier of the multidecadal signal [15] , [20] . Contrary to this view, it has also been suggested that multidecadal climate oscillations, including the AMO, are driven by cyclic variations in solar activity [21] , [22] . This controversy has been fuelled by difficulties in resolving the spectral behaviour of the AMO. Here, we show, based on spectral analyses of high-resolution climate proxy records from the region bounding the North Atlantic, that distinct ∼ 55- to 70-year oscillations characterized the North Atlantic ocean-atmosphere variability over the past 8,000 years. Moreover, through comparisons between proxy records and instrumental data, we investigate the linkage between these Holocene multidecadal climate oscillations and the modern AMO. We also test solar variability as a possible forcing mechanism underlying this climate variability. Linking the AMO to climate proxy data Several studies have linked precipitation changes to AMO variability [7] , [9] , [10] , but the coupling between the AMO and precipitation anomalies is spatially complex; a warm AMO phase is thought to be associated with a positive precipitation anomaly in the Sahel region of Africa, whereas precipitation anomalies in, for example, Mexico appear to have been in anti-phase with the AMO and Sahel precipitation [7] . 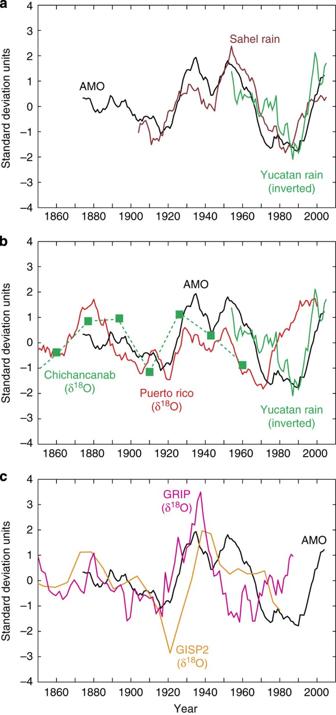Figure 2: Linking Holocene climate records to the AMO index. (a) The Atlantic multidecadal oscillation (AMO) index4(black) shown together with instrumental records of precipitation variability in the Sahel region (brown) and on the Yucatan peninsula (green; courtesy of the National Meteorological Survey of Mexico). Note that the instrumental precipitation record from the Yucatan peninsula has been inverted, implying that warm (cold) AMO phases correspond to dry (wet) conditions. (b) The AMO index4(black) and the instrumental precipitation record from the Yucantan peninsula (green) is shown together with the coral-based δ18O record from Puerto Rico14(red) and the δ18O record from lake Chichancanab29(dashed green line). Note that the sign of the Chichancanab record (high δ18O=dry) means that warm AMO phases were associated with drier conditions, which is in full agreement with the instrumental record from the Yucatan peninsula and numerical model simulations7. (c) The AMO index4(black) along with the δ18O records from GRIP24(magenta) and GISP226(orange) ice cores. All the records have been detrended and normalized to one standard deviation unit. Nine-year running means were computed for all records with an annual resolution, that is, the instrumental records and the δ18O record from Puerto Rico, whereas 20-year running means were computed for the GRIP and GISP2 δ18O records to suppress short-term δ18O scatter. This is illustrated in Figure 2 , which compares the AMO index to instrumental data and climate proxy records from the Atlantic region. Recent model experiments, however, have failed to identify the AMO as the primary driver of recent reductions in Sahel rainfall [23] . In fact, these model simulations indicate that the major climate impacts of multidecadal changes in Atlantic Ocean SST over land are to be found in North America and the northern part of South America. To investigate the existence and origin of the AMO on Holocene timescales, we carefully selected seven Holocene climate proxy records from the North Atlantic region, including five ice-core records from Greenland [24] , [25] , [26] , [27] and the Canadian Arctic [28] , one lacustrine record from the Yucatan peninsula [29] , Mexico, and a marine record from the Cariaco Basin [30] , north of Venezuela ( Figs 3 and 4 ). These records derive from sites that are located close to the current summer positions of the atmospheric polar front (PF) or the intertropical convergence zone (ITCZ). The records were chosen based on a their documented sensitivity to variations in North Atlantic SST, and an average temporal resolution of 25 years or better ( Supplementary Table S1 ) over a time span of 8,000 years or more. The majority of these climate proxy records overlap the instrumental AMO record in time, and, although the temporal resolution for some of the proxy records is relatively low for the past 140 years, they clearly tend to co-vary with the AMO index ( Fig. 2 ). The precipitation proxy record from Lake Chichancanab (Yucatan) co-varies with both the AMO index and a coral-based SST reconstruction from Puerto Rico, with the instrumental precipitation record from the Yucatan peninsula looking almost like an extension of the Lake Chichancanab proxy record ( Fig. 2b ). The comparisons show that warm AMO phases correlate with dry periods on the Yucatan Peninsula, which is in accord with numerical model simulations [7] (note that the instrumental rainfall record from Yucantan has been inverted in Fig. 2b, and that high δ 18 O values from Lake Chichancanab correspond to dry periods). The GRIP record and, in particular, the GISP2 record also co-vary with the AMO index over the last 140 years ( Fig. 2c ), suggesting that the two ice-core records were sensitive to North Atlantic SST variations, with increasing SST leading to increasing δ 18 O values as expected. Apart from North Atlantic SST variations, climate variability observed in these proxy records may to some extent also have been driven by other Northern Hemisphere (NH), or even global-scale, climate effects that are correlated with the AMO. The potential existence of such NH teleconnections is underpinned by coupled ocean-atmosphere models [5] , [20] . Irrespective of this ambiguity regarding the principal driving mechanism, it remains very likely that the observed multidecadal variability, be it directly or indirectly, reflects North Atlantic SST variations related to the AMO. Figure 2: Linking Holocene climate records to the AMO index. ( a ) The Atlantic multidecadal oscillation (AMO) index [4] (black) shown together with instrumental records of precipitation variability in the Sahel region (brown) and on the Yucatan peninsula (green; courtesy of the National Meteorological Survey of Mexico). Note that the instrumental precipitation record from the Yucatan peninsula has been inverted, implying that warm (cold) AMO phases correspond to dry (wet) conditions. ( b ) The AMO index [4] (black) and the instrumental precipitation record from the Yucantan peninsula (green) is shown together with the coral-based δ 18 O record from Puerto Rico [14] (red) and the δ 18 O record from lake Chichancanab [29] (dashed green line). Note that the sign of the Chichancanab record (high δ 18 O=dry) means that warm AMO phases were associated with drier conditions, which is in full agreement with the instrumental record from the Yucatan peninsula and numerical model simulations [7] . ( c ) The AMO index [4] (black) along with the δ 18 O records from GRIP [24] (magenta) and GISP2 [26] (orange) ice cores. All the records have been detrended and normalized to one standard deviation unit. Nine-year running means were computed for all records with an annual resolution, that is, the instrumental records and the δ 18 O record from Puerto Rico, whereas 20-year running means were computed for the GRIP and GISP2 δ 18 O records to suppress short-term δ 18 O scatter. 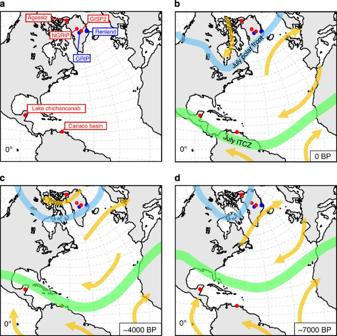Figure 3: Location of the climate proxy records and schematic overview of the major atmospheric systems. (a) Location of proxy records used in this study. Red dots signify records for which results of the spectral analyses are included inFigure 5. For records marked with blue circles we refer toSupplementary Figures S5 and S8. (b) Modern atmospheric systems of the North Atlantic region. Not taking multi-centennial climate variations into account, our study indicates that this scenario may also represent average conditions for the period 0–3,000 years BP, where an overall 'neo-glacial' regime with more frequent meridional atmospheric circulation patterns and an ITCZ located close to the Cariaco site during Northern Hemisphere (NH) summer was prevalent. (c)∼4,000 years BP: solar insolation was higher than present in the NH, but lower in the Southern Hemisphere (SH). Both the ITCZ and the atmospheric polar front were generally located north of its present position during the NH summer, and a zonal atmospheric circulation dominated. The position of the summer PF over Greenland was, however, roughly similar to the present location. (d)∼7,000 years BP: significantly higher NH summer insolation than today, whereas it was lower in the SH (opposite in winter). The ITCZ was located north of its present position, with the PF also displaced well to the north in the North Atlantic sector, but, at least initially, less so in the N. American/Canadian sector, where the last remains of the Laurentide Ice Sheet (white zone) were still present in the Baffin Land region (until∼7,000 years BP). These conditions may be representative for the average conditions between 6,000 and 8,000 BP. PF, atmospheric polar front; ITCZ, intertropical convergence zone. The yellow arrows indicate the dominant wind directions. Full size image Figure 3: Location of the climate proxy records and schematic overview of the major atmospheric systems. ( a ) Location of proxy records used in this study. Red dots signify records for which results of the spectral analyses are included in Figure 5 . 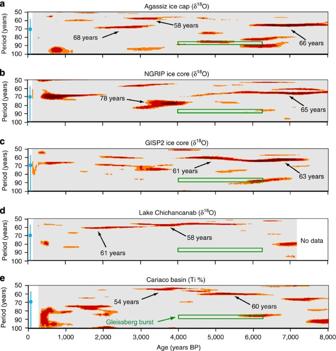Figure 5: Multidecadal climate oscillations in the region bounding the North Atlantic Ocean. (a) Spectrogram delineating the temporal distribution of highly significant (orange:χ2>90%, red:χ2>95%, and dark red:χ2>99%) spectral power of the δ18O record from the Agassiz ice cap28. Distributions of highly significant spectral power are also shown for (b) the NGRIP δ18O record27, (c) the GISP2 δ18O record26, (d) the Lake Chichancanab δ18O record29, and (e) the Ti (%) record from the Cariaco Basin30. For this spectral analysis, the data were grouped in overlapping 2,000-year windows, with a spacing of 50 years, for the interval 1,000–8,000 BP. Spectral estimates for the last 1,000 years were obtained by decreasing the window size linearly from 2,000 years at 1,000 BP to 200 years at 100 BP in steps of 25 years. Only the 50- to 100-year period range is shown, because this encompasses the AMO range normally reported in the literature. The blue circle denotes the spectral peak for the instrumental AMO record, whereas the blue line shows the associated uncertainty. The green rectangles delineate the prominent burst in intensity of the Gleissberg (∼88 year) solar cycle between 4,000 and 6,250 BP34. For records marked with blue circles we refer to Supplementary Figures S5 and S8 . ( b ) Modern atmospheric systems of the North Atlantic region. Not taking multi-centennial climate variations into account, our study indicates that this scenario may also represent average conditions for the period 0–3,000 years BP, where an overall 'neo-glacial' regime with more frequent meridional atmospheric circulation patterns and an ITCZ located close to the Cariaco site during Northern Hemisphere (NH) summer was prevalent. ( c ) ∼ 4,000 years BP: solar insolation was higher than present in the NH, but lower in the Southern Hemisphere (SH). Both the ITCZ and the atmospheric polar front were generally located north of its present position during the NH summer, and a zonal atmospheric circulation dominated. The position of the summer PF over Greenland was, however, roughly similar to the present location. ( d ) ∼ 7,000 years BP: significantly higher NH summer insolation than today, whereas it was lower in the SH (opposite in winter). The ITCZ was located north of its present position, with the PF also displaced well to the north in the North Atlantic sector, but, at least initially, less so in the N. American/Canadian sector, where the last remains of the Laurentide Ice Sheet (white zone) were still present in the Baffin Land region (until ∼ 7,000 years BP). These conditions may be representative for the average conditions between 6,000 and 8,000 BP. PF, atmospheric polar front; ITCZ, intertropical convergence zone. 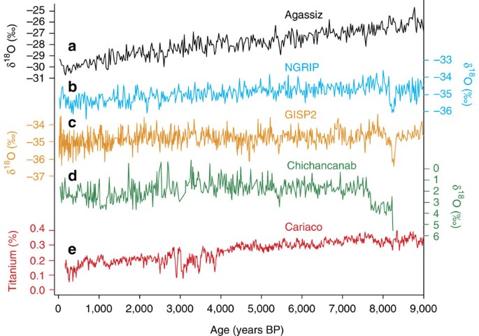The yellow arrows indicate the dominant wind directions. Figure 4: High-resolution Holocene climate proxy records from the region bounding the North Atlantic Ocean. Oxygen isotope (δ18O) records from (a) the Agassiz ice cap28(b) the NGRIP ice core27(c) the GISP2 ice core26and (d) Lake Chichancanab29. (e) Titanium (%) record from the Cariaco Basin30. The curves show the original data with no filtering or detrending applied. Full size image Figure 4: High-resolution Holocene climate proxy records from the region bounding the North Atlantic Ocean. Oxygen isotope (δ 18 O) records from ( a ) the Agassiz ice cap [28] ( b ) the NGRIP ice core [27] ( c ) the GISP2 ice core [26] and ( d ) Lake Chichancanab [29] . ( e ) Titanium (%) record from the Cariaco Basin [30] . The curves show the original data with no filtering or detrending applied. Full size image Spectral pattern of the Holocene North Atlantic climate By applying the Lomb-Scargle Fourier transform [31] and a 2,000-year running-window approach to each climate proxy record, we calculated the spectral density distributions, from which red-noise false-alarm levels [31] were estimated and colour-coded. This novel combination of methods allows not only a detailed assessment of temporal variations in the cyclic behaviour of unevenly spaced data, but also a clear distinction between temporal distributions of, for example, ∼ 60-, 70- and 80-year oscillations. One major advantage of using the Lomb-Scargle Fourier transform is that it enables computation of spectral significances without having to interpolate the data onto a common time step. All records display a relatively narrow, dominant oscillation band between ∼ 55 and 70 years, as well as weaker oscillations scattered around the 70- to 125-year band. Significant spectral power overlapping the ∼ 88-year Gleissberg solar activity band is also observed for some of the studied records, most notably the Agassiz and GISP2 δ 18 O records ( Fig. 5a,c ), but it is only observed in discrete intervals and generally dwarfed by the spectral power observed in the 55- to 70-year band. Spectral estimates for the last 1,000 years are established by gradual narrowing of the time window, which by definition gives rise to gradual spectral blurring towards the near-present, where the oscillation bands widen. The fact that the dominant 55- to 70-year oscillation in these Holocene records is based on climate proxies, which co-vary with the AMO index over the last 140 years, have the expected sign, and which resemble the oscillations inferred from both the AMO index and model studies of SST variations, clearly indicate that this quasi-periodic oscillation reflects the Holocene AMO behaviour. This observation is in close agreement with a coral-based reconstruction of Caribbean SST variations over the past 250 years [14] , which shows a clear 60-year oscillation ( Supplementary Fig. S1 ), and it is consistent with the approximately 60-year variability observed in a 1,000-year control integration of a coupled ocean-atmosphere model [15] . It is noticeable that the multidecadal variability related to the AMO in some records, particularly those from central Greenland, appears to be the dominant climate variability throughout the last 8,000 years, that is, the amplitude of the long-term trends is comparable to or smaller than the multidecadal-scale variability ( Fig. 4 ). Figure 5: Multidecadal climate oscillations in the region bounding the North Atlantic Ocean. ( a ) Spectrogram delineating the temporal distribution of highly significant (orange: χ 2 >90%, red: χ 2 >95%, and dark red: χ 2 >99%) spectral power of the δ 18 O record from the Agassiz ice cap [28] . Distributions of highly significant spectral power are also shown for ( b ) the NGRIP δ 18 O record [27] , ( c ) the GISP2 δ 18 O record [26] , ( d ) the Lake Chichancanab δ 18 O record [29] , and ( e ) the Ti (%) record from the Cariaco Basin [30] . For this spectral analysis, the data were grouped in overlapping 2,000-year windows, with a spacing of 50 years, for the interval 1,000–8,000 BP. Spectral estimates for the last 1,000 years were obtained by decreasing the window size linearly from 2,000 years at 1,000 BP to 200 years at 100 BP in steps of 25 years. Only the 50- to 100-year period range is shown, because this encompasses the AMO range normally reported in the literature. The blue circle denotes the spectral peak for the instrumental AMO record, whereas the blue line shows the associated uncertainty. The green rectangles delineate the prominent burst in intensity of the Gleissberg ( ∼ 88 year) solar cycle between 4,000 and 6,250 BP [34] . Full size image The Holocene AMO signal appears to have been quasi-periodic and the associated climate response to have been of highly variable intensity, both in time and space. In the tropical Atlantic, especially at Lake Chichancanab, the AMO response signal was generally relatively weak during the NH warming of the Holocene thermal maximum (HTM) between 5,500 and 9,000 BP, after which it picked up in intensity ( Fig. 5 and Supplementary Figs S2 and S3 ). The Arctic ice-core records reveal a different response pattern, as they indicate that the Arctic AMO signal was strongest during the HTM, after which the intensity of the Arctic AMO response generally faded, albeit only to reappear in sudden bursts, most notably around 3,000 BP ( Fig. 5 and Supplementary Figs S4-S8 ). Interestingly, the northernmost sites (Agassiz and NGRIP) seem to have the earliest AMO response peak (6,000–8,000 years BP) with a delayed peak at GISP2 and GRIP (4,500–7,000 years BP). The most notable exception from this pattern is the Renland ice-core record ( Supplementary Fig. S8 ), which, similar to the tropical records, shows little sign of an AMO response signal during the HTM, but a strong signal from around 3,500 BP onwards. This discrepancy may be due to the fact that the Renland δ 18 O-signal was influenced by the 'local' coastal setting, characterized by more widespread HTM melting and maritime climate conditions that significantly differed from the environment found in the central, high-altitude part of the ice cap. Through the past 8,000 years, minor shifts appear to have occurred in the dominating period within the 55- to 70-year band ( Fig. 5 ). The dominant oscillation period in the interval of 5,500–8,000 BP was ∼ 65 years, whereas it shortened somewhat between 5,500 BP and ∼ 2,700 BP (55–60 years). The period of the dominant oscillations increased slightly again after ∼ 2,700 BP (65–70 years), but the oscillations were generally not as well defined as during the early Holocene, when the AMO period bandwidth appears to have been narrower. The role of the Gleissberg solar cycle To investigate whether these Holocene 55- to 70-year climate oscillations could have been a direct response to cyclic changes in solar activity, we searched for evidence of an ∼ 60-year cycle in two Holocene solar activity reconstructions based on 14 C from the IntCal04 radiocarbon calibration curve [32] and 10 Be from the GRIP ice core [33] . Spectral analyses of both solar reconstructions show that the Gleissberg cycle ( ∼ 88 years) was very prominent between 4,000 and 6,250 years BP and became remarkably vague from ∼ 3,500 years BP onwards [34] . This ' Gleissberg burst ' represents the most dominant oscillation in this frequency range of both solar spectra. There is no substantial evidence for an ∼ 60-year oscillation in the solar reconstruction based on 14 C, whereas the 10 Be-based reconstruction shows some evidence of such an oscillation between 1,600–2,300 BP ( Supplementary Figs S9 and S10 ). The origin of this ∼ 60-year oscillation in the 10 Be reconstruction is therefore unknown, but it could reflect non-solar cyclic changes in the beryllium transport path that influenced the deposition rate over Greenland. Solar forcing is therefore not likely to be responsible for the dominant 55- to 70-year Holocene AMO pattern, which implies that the Holocene AMO pattern more likely reflects internal, quasi-periodic variability in Atlantic Ocean circulation, in accordance with, for example, the HadCM3 model [20] . The coupling from the AMO to regional climate conditions cannot be expected to be constant in time; we would expect north-south migrations of the ITCZ and atmospheric PF to be prime modulators of this coupling. The decrease in NH summer insolation is known to have been accompanied by a southward migration of the ITCZ [30] , a general change in the atmospheric circulation [35] , including a southward shift of the jet stream and Icelandic Low [36] as well as a major change in the Atlantic Meridional overturning circulation [37] . Accordingly, the AMO response signal in the records studied seems to exhibit a general shift in its pattern within the last 8,000 years, as the signal was most pronounced in the Arctic during the HTM, whereas in the tropics its maximum was generally reached after the HTM. Moreover, coeval with these large-scale changes, minor shifts in the dominant frequency occurred. We hypothesize that this overall pattern is a consequence of large-scale circulation changes driven by orbitally-induced changes in insolation. Thus, during the HTM, a northwardly displaced and highly zonally arranged atmospheric circulation pattern [38] led to minimum sea-ice cover in the Arctic [39] , which allowed a much stronger ocean-atmosphere interaction compared with times characterised by a widespread presence of sea ice. In contrast, conditions in the tropics were more stable during the HTM, which may be attributed to a more northerly location of the ITCZ, implying that the tropical sites were situated outside the range of the annual ITCZ migratory precipitation belt ( Fig. 3d ). We propose that the subsequent southward migration of the ITCZ during the mid to late Holocene [30] , and the associated southward movement of the PF and increase in Arctic sea-ice cover [39] , implied that the high-Arctic sites were now situated more permanently north of the atmospheric PF and outside the immediate reach of SST-controlled multidecadal variations in atmospheric circulation. This hypothesis is consistent with the observation that the prominent and well-resolved ∼ 65-year oscillation terminates first in the record from the Agassiz ice cap, the most northerly site ( Fig. 5 ). Towards the end of the HTM (5,500–6,000 BP), as the ITCZ moved southward and closer to the tropical sites ( Fig. 3c ), these sites seem to have become more sensitive to changes in ITCZ, and hence the AMO, as even slight changes in North Atlantic SST can cause N-S shifts in the ITCZ and thus in rainfall [19] . Between 2,000 and 3,500 BP there was a statistically significant recurrence of multidecadal oscillations in the Arctic. This interval overlaps with a part of the neo-glaciation between 2,000 and 3,000 BP, which was characterized by relatively high SST and generally warmer, and particularly unstable, climate conditions in parts of the northern North Atlantic region [40] . Such conditions meant that the Arctic sites temporarily became more sensitive to multidecadal SST oscillations, possibly due to an associated reduction in Arctic sea-ice cover. However, the major changes in North Atlantic Ocean [41] , [42] , [43] and atmospheric circulation patterns that followed the neo-glaciation in both hemispheres [44] , [45] , [46] led to a generally weakened, and probably less coherent, AMO response signal after ∼ 2,000 BP. This change was accompanied by a distinct SST decline between 2,000 and 500 BP in some parts of the northern North Atlantic [40] . The most pronounced AMO signal observed after 2,000 BP is found in the records from central Greenland, possibly because a position of the summer PF relatively close to these ice-core sites meant that they were somewhat sensitive to the AMO through its influence on the PF. In general, the episodes characterized by an increased strength of the AMO signal in the Arctic records after ∼ 3,500 BP may be attributed to minor shifts in the summer PF, which most likely was located relatively close to the ice-core sites in central Greenland throughout this interval ( Fig. 3b ). This new hypothesis, linking regional-scale AMO response patterns to insolation-driven migration of the ITCZ and PF, calls for further study using coupled ocean-atmosphere models and new high-resolution proxy records. A quasi-persistent 55- to 70-year oscillation thus appears to have influenced climate in the North Atlantic region during both warmer and colder intervals. Underpinned by comparative studies of instrumental and proxy climate records, we infer that these Holocene climate variations correspond to the AMO recognized in instrumental data. The AMO known from the relatively short instrumental record therefore appears, when viewed over longer time intervals, to display a more well-defined and slightly narrower oscillation band than previously believed. Hence, our findings suggest that a 55- to 70-year quasi-persistent AMO, forced by internal ocean-atmosphere variability, existed throughout most of the Holocene. Its coupling to regional climate appears to have been modulated by insolation-driven shifts in atmospheric circulation patterns and sea-ice cover. These findings underline the need to better understand the influence of the AMO on global and regional climate variations over the last century. The study has also implications for future climate scenarios, as our analyses suggest that the AMO exerted a stronger influence on regional climate variability in the northern North Atlantic region during times of high North Atlantic SST compared with colder periods. Given the increase in North Atlantic SST over the past ∼ 30 years, and the expected future increase in global SST, we anticipate that the influence of the AMO on climate variability in the northern North Atlantic region will increase in response to the future warming of the North Atlantic Ocean. Moreover, the AMO shifted into its warm phase in the 1990s ( Fig. 1 ), which may have accentuated global warming in this period. A return from a warm to a cold AMO phase could temporarily mask the effects of anthropogenic global warming [47] , and thus lead to possible underestimation of future warming if the variability of the AMO is not taken into account. Selection of key North Atlantic climate proxy records Altogether seven climate proxy records were analysed in this study, including (i) five Arctic ice-core records from Greenland [24] , [25] , [26] , [27] and Canada [28] , and (ii) two tropical records; a lacustrine record from the Yucatan peninsula [29] in Mexico and a marine record from the Cariaco Basin [30] north of Venezuela. The records were chosen based on two selection criteria: (i) their documented sensitivity to subtle variations in North Atlantic SST, and (ii) an average temporal resolution of 25 years or better over a time span of 8,000 years or more. The data from the Ellesmere Island Agassiz ice cap [28] and Greenland ice cores [24] , [25] , [26] , [27] recorded precipitation variability at high northern latitudes, reflecting the tracks of extra-tropical cyclones and stability of the Greenland semi-permanent high-pressure cell under influence of changes in the Northern Annual Mode. Advection of Atlantic moisture towards central Greenland is mainly controlled by winds from a south-easterly direction that occur along the northern flank of North Atlantic cyclones [48] . A positive correlation has been shown between warm AMO phases and temperatures in Greenland and eastern Canada [7] . The two sites located in the Caribbean region are presently situated at the northern boundary of the summer (July) ITCZ, which implies a well-defined summer precipitation regime [38] . Although the Chichancanab record [29] is representative of variations in precipitation on a more local scale, the Cariaco precipitation record [30] shows the effect of riverine run-off from northeast South America on a more regional scale. Sea-surface salinities from the Caribbean and Mexican Gulf show a strong connection with North Atlantic SST [14] , [49] with less (more) saline conditions in the tropics coinciding with warmer (cooler) North Atlantic SSTs, and thus with stronger (weaker) overturning circulation [14] . Several other records that potentially are relevant to this study exist, including a high-resolution study of variations in SST based on alkenones from marine core MD99-2275 north of Iceland [50] . Unfortunately, this record covers only the past 4,500 years and so cannot be used to study multidecadal oscillation throughout the Holocene, but it does show the presence of highly significant 50- to 70-year oscillations ( Supplementary Fig. S11 ). The speleothem δ 18 O record from Crag Cave [51] , Ireland, does cover the past 10,000 years, but the sampling is too irregular to reliably resolve 50- to 100-year periods uniformly through the Holocene. Other relevant high-resolution records (δ 18 O, δ 13 C, Mg/Ca) derive from estuarine sediments in Chesapeake Bay, eastern USA, which span the last 2,000 years and the interval 6,000–7,000 BP [52] . All proxy records from the interval 6,000–7,000 BP show significant multidecadal variability centred at ∼ 60, 40 and 20 years, whereas the multidecadal variability over the last 2,000 years was confined to the ∼ 20- to 40-year timescale. This is consistent with the pattern observed in our study in the sense that the ∼ 60-year oscillation generally seems to have been less prominent during the past 2,000 years compared with earlier parts of the Holocene. Spectral density distributions To be able to resolve the temporal distribution of climate cyclicities with almost similar periods (such as ∼ 60, 70 and 80 years) in the climate proxy records, we used a novel approach to determine spectral density distributions for unevenly spaced data based on a well-known and widely used method. The climate proxy records were first detrended to suppress spectral leakage from the low-frequency harmonics ( ∼ 1,000 year and longer periods). Subsequently, we grouped the data in overlapping 2,000-year windows, with a spacing of 50 years, before calculating the spectrum and associated red-noise false-alarm levels [31] for all individual windows. A window size of ∼ 2,000 years was chosen to obtain optimal balance between spectral smoothing and temporal resolution (in this study the degree of spectral smoothing depends solely on the window size). Spectral estimates for the last 1,000 years were obtained by decreasing the window size linearly from 2,000 years at 1,000 BP to 200 years at 100 BP in steps of 25 years. Note that this gradual narrowing of the window size is by definition accompanied by a gradual blurring of the spectral resolution. Thus, we should not expect the fine spectral lineaments to be resolved all the way to the present day. The spectrum associated with each data window was estimated using the Lomb-Scargle Fourier transform [53] , [54] for unevenly spaced data and one Welch-type window. Similar to the more traditional Fourier analysis, the Lomb-Scargle method is based on a least-squares fit of sinusoids to the time series data. The Lomb-Scargle transform has been widely used to study climate oscillations, because this method does not require that unevenly spaced time series data are interpolated onto an equidistant timescale. Red-noise model and statistical significances The univariate spectra were bias-corrected using 1,000 Monte Carlo simulations. This was carried out by use of the publicly available REDFIT program [31] , [55] , which automatically produces first-order autoregressive (AR1) time series with sampling times and characteristic timescales matching those of the real climate data. To assess the statistical significance of a spectral peak, REDFIT estimates the upper confidence interval of the AR1 noise for various significance levels based on a χ 2 distribution [31] . This approach has been widely used in other palaeoclimatological studies to evaluate the significance of spectral peaks [56] , [57] . In this study, we aligned all the individual spectra, based on data grouped in time windows with a spacing of 50 years (25 years for the interval 0–1,000 BP), according to their age, given by the midpoint of the time window, and coloured-coded the frequencies for which the spectral power exceeded red-noise false-alarm levels ( ∼ confidence levels) of 90, 95 and 99%. Standard tests [31] showed that the climate data series could in fact be approximated sufficient well by an AR1 model, on which the accuracy of the estimated red-noise false-alarm levels depends. Finally, we also ensured that the temporal distribution of spectral significance was insensitive to the detrending method applied, by for example, repeating the whole process using alternative detrending methods. How to cite this article: Knudsen, M. F. et al . Tracking the Atlantic Multidecadal Oscillation through the last 8,000 years. Nat. Commun. 2:178 doi: 10.1038/ncomms1186 (2011).